Histone deacetylation promotes mouse neural induction by restricting Nodal-dependent mesendoderm fate Cell fate determination requires the cooperation between extrinsic signals and intrinsic molecules including transcription factors as well as epigenetic regulators. Nevertheless, how neural fate commitment is regulated by epigenetic modifications remains largely unclear. Here we show that transient histone deacetylation at epiblast stage promotes neural differentiation of mouse embryonic stem cells (mESCs). Histone deacetylase 1 ( HDAC1 ) deficiency in mESCs partially phenocopies the inhibition of histone deacetylation in vitro , and displays reduced incorporation into neural tissues in chimeric mouse embryos in vivo . Mechanistic studies show that Nodal , which is repressed by histone deacetylation, is a direct target of HDAC1. Furthermore, the inhibition of histone deacetylation in the anterior explant of mouse embryos at E7.0 leads to Nodal activation and neural development repression. Thus, our study reveals an intrinsic mechanism that epigenetic histone deacetylation ensures neural fate commitment by restricting Nodal signalling in murine anterior epiblast ex vivo and mESC in vitro . The lineage specification of three germ layers occurs during gastrulation, an important event during early embryogenesis [1] , [2] . Posterior epiblast cells ingress through the primitive streak to generate mesoderm and endoderm, and the cells that remain in the anterior epiblast give rise to neuroectoderm [1] . The formation of the neuroectoderm, termed neural induction, is the first step in the development of the central nervous system and initiates at approximately embryonic day (E) 7.5 [2] , [3] . The inhibition of extrinsic signals such as BMPs, WNTs and Nodal in the prospective neuroectoderm is imperative for the appropriate neural fate commitment [4] . Nevertheless, the mechanisms underlying intrinsic programmes, especially epigenetic modifications, that participate in the neural induction remain largely unclear. Early studies on neural induction primarily focused on extrinsic signals. The Nodal signalling pathway plays a crucial role in proximal–distal and anterior–posterior (A–P) axis patterning of the epiblast [1] , [3] , [5] , [6] , [7] . Nodal is expressed in the posterior region of the early mouse embryo to promote the formation of primitive streak and mesendoderm development. The Nodal antagonists Cer1 and Lefty1, which are primarily expressed in anterior visceral endoderm, endow the anterior epiblast neural fate and block the mesendoderm lineage commitment. In Nodal −/− embryos, neural specification occurs precociously with the expansion of the neural plate; however, the mesoderm and the endoderm fail to form [8] , [9] , [10] . In contrast, C er1 and Lefty1 double mutants exhibit enlarged mesoderm and compromised neuroectoderm [11] . Clearly, Nodal signalling must be controlled delicately for the appropriate determination of neuroectoderm and mesendoderm identities. Recent studies have revealed that in addition to the extrinsic signals, intrinsic programmes mediated by transcription factors and epigenetic regulators play important roles in neural fate determination. Several transcription factors such as Zic2, Otx2, Pou3f1, Sox2 and Zfp521 promote neural fate commitment in a cell-autonomous manner [12] , [13] , [14] . Our studies and others have also shown that histone demethylase Kdm7a, an epigenetic regulator, is required for the neural differentiation of mouse embryonic stem cells (mESCs) in vitro and in chick and zebrafish embryos in vivo [15] , [16] , [17] . However, it remains largely unknown whether other epigenetic modifications, such as histone acetylation/deacetylation, participate in the neural induction. Histone deacetylases (HDACs) inhibit gene expression by removing acetyl groups from crucial lysine residues of histone proteins. There are four classes of HDACs in mammals: HDAC1–3 and HDAC8 in class 1; HDAC4–7, HDAC9 and HDAC10 in class 2; sirtuins in class 3; and HDAC11 in class 4 (ref. 18 ). Trichostatin A (TSA) and sodium butyrate (NaB) are identified as HDAC inhibitors (HDACi) that repress both class I and II HDACs [19] , [20] . HDACs are involved in the development of epidermis [21] , heart [22] and pancreas [23] and the specification of oligodendrocytes [24] , [25] , neurons [26] , adipocytes [27] , osteoblasts [28] and T-cells [29] , as well as the self-renewal of ESCs and the reprogramming process of induced pluripotent stem cells [30] , [31] . HDAC1 is highly expressed in the head fold and the neural fold at E8.5, and HDAC1 -null mutant mouse is lethal before E10.5 with abnormal head formation [32] . Deletion of HDAC1 and HDAC2 in neural progenitor cells (NPCs) with Gfap-Cre or Nestin-Cre leads to abnormal neurogenesis, a relatively late event in brain development [33] , [34] . Nonetheless, whether and how epigenetic modifications such as histone deacetylation mediated by HDACs participate in mouse neural fate commitment is little known. The in vitro neural differentiation of mESCs and epiblast stem cells (EpiSCs) recapitulates the step-wise events of early neural development in vivo and also provides approaches to investigate the fundamental regulatory mechanisms of neural induction [35] , [36] , [37] , [38] , [39] , [40] , [41] . Our previous study showed that similar to the neural fate commitment in the mouse embryo in vivo , two stages occur during mESC neural differentiation in vitro : one stage from mESCs to EpiSCs, and the other stage from EpiSCs to NPCs. In addition, neural fate determination occurs in the latter stage [42] . In this study, we reveal that the transient histone deacetylation at the epiblast-like stage is essential for mESC neural fate determination in vitro . HDAC1 deficiency in mESCs partially phenocopies the inhibition of histone deacetylation in vitro , and displays reduced incorporation into neural tissues in chimeric mouse embryos in vivo . The inhibition of histone deacetylation in the anterior epiblast at E7.0 ex vivo impairs neural fate commitment and enhances mesendoderm development. We further uncover a novel molecular mechanism of neural induction that histone deacetylation, an essential epigenetic regulation, ensures neural fate commitment primarily by repressing extracellular Nodal signalling. Transient histone deacetylation in mESC neural commitment In this study, we utilized the mESC line 46C, in which the expression of green fluorescent protein (GFP) was driven by the endogenous Sox1 gene (Sox1–GFP), to neural differentiation in a monolayer manner as previously described [43] . The expression of epiblast-specific markers (Oct4, Fgf5, Claudin6 and Otx2) was detected in epiblast-like day 2 cells, displaying a high nuclear-cytoplasm ratio ( Fig. 1a , Supplementary Fig. 1 ). GFP + and Pax6 + NPCs were readily observed at the differentiation day 4 and day 6 ( Fig. 1a,b ). Quantified data revealed that the percentage of GFP + NPCs was ∼ 30% at day 4 and was increased to 70% at day 6 ( Fig. 1b ). Quantitative PCR (qPCR) assays showed that on differentiation, the expression of the pluripotency genes Oct4 and Rex1 decreased, and Fgf5 expression increased sharply at day 1 and remained high from day 2 to day 3, and diminished thereafter ( Fig. 1c ). The expression of the early anterior neuroectoderm marker Zic2 increased at day 1 and reached the peak at day 3, and the expression of the NPC markers Sox1 and Pax6 was readily detected after day 4 ( Fig. 1d ). Clearly, the neural differentiation of the 46C cells proceeded through multiple stages: ESC stage, Oct4 + /Fgf5 + epiblast-like stage at day 2 and Sox1–GFP + NPCs stage at day 4–6, implicating that mESC neural differentiation recapitulates the sequential cell fate changes of neural development in vivo . To determine whether histone acetylation/deacetylation is associated with mESC neural differentiation, western blotting was performed to examine the acetylation levels of histone H3. Comparing with that in the undifferentiated mESCs, the acetylation of histone H3 at both lysine 9 (H3K9ac) and the N terminus (H3ac) declined markedly at the onset of neural differentiation, remained at low levels until day 3, and was restored to high levels by day 4–6 ( Fig. 1e ). The results above show that a transient histone deacetylation event occurs at the epiblast-like stage during mESC neural differentiation. 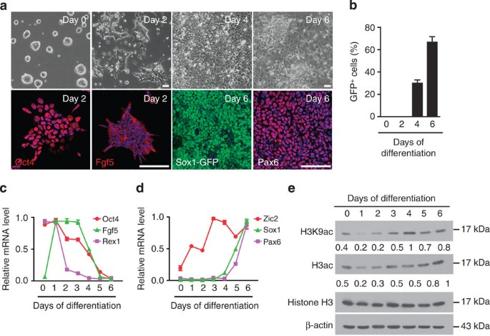Figure 1: The dynamic pattern of histone H3 acetylation levels during mESC neural differentiation. (a) Representative cellular morphologies during 46C neural differentiation from four independent experiments. 46C cells were plated in N2B27 medium and differentiated for 6 days. Images of undifferentiated 46C, phase contrast and immunocytochemistry for Oct4 and Fgf5 in day 2 cells, phase contrast of day 4 and day 6 cells, Sox1–GFP expression and immunocytochemistry for Pax6 of day 6 cells were shown. Nuclei were stained with DAPI. Scale bar, 75 μm. (b) Statistical analysis of Sox1–GFP+cells during 6 days of neural differentiation (n=4). (c) Gene expression analysis during 6 days of neural differentiation. Oct4, Rex1, ESC marker; Fgf5, epiblast marker. Relative gene expression levels were normalized to the expression ofgapdh. (d) Gene expression analysis during 6 days of neural differentiation. Zic2, early neuroectoderm marker; Sox1, Pax6, definitive NPC marker. Relative gene expression levels were normalized to the expression ofgapdh. (e) Western blotting analysis of H3ac and H3K9ac levels during mESC neural differentiation. The data inc,dwere shown from three independent experiments. Data inb–drepresent mean±s.d. *P<0.05, Student’st-test. Figure 1: The dynamic pattern of histone H3 acetylation levels during mESC neural differentiation. ( a ) Representative cellular morphologies during 46C neural differentiation from four independent experiments. 46C cells were plated in N2B27 medium and differentiated for 6 days. Images of undifferentiated 46C, phase contrast and immunocytochemistry for Oct4 and Fgf5 in day 2 cells, phase contrast of day 4 and day 6 cells, Sox1–GFP expression and immunocytochemistry for Pax6 of day 6 cells were shown. Nuclei were stained with DAPI. Scale bar, 75 μm. ( b ) Statistical analysis of Sox1–GFP + cells during 6 days of neural differentiation ( n =4). ( c ) Gene expression analysis during 6 days of neural differentiation. Oct4, Rex1, ESC marker; Fgf5, epiblast marker. Relative gene expression levels were normalized to the expression of gapdh . ( d ) Gene expression analysis during 6 days of neural differentiation. Zic2, early neuroectoderm marker; Sox1, Pax6, definitive NPC marker. Relative gene expression levels were normalized to the expression of gapdh . ( e ) Western blotting analysis of H3ac and H3K9ac levels during mESC neural differentiation. The data in c , d were shown from three independent experiments. Data in b – d represent mean±s.d. * P <0.05, Student’s t -test. Full size image Histone deacetylation promotes mESC neural commitment To investigate whether histone deacetylation plays an essential role in mESC neural differentiation, TSA (HDACi) was added at day 2 of the epiblast-like stage for 24 h, and the percentage of GFP + NPCs was quantified at day 6. TSA treatment inhibited mESC neural differentiation in a dose-dependent manner ( Fig. 2a ). To avoid the apoptosis and cell cycle arrest caused by the high concentration of TSA, 10 nM TSA was used in our study as previously reported [30] . As expected, 10 nM TSA treatment efficiently blocked histone deacetylation, and the acetylation level of H3 in TSA-treated cells was much higher than that in the DMSO-treated control cells at day 3 ( Fig. 2b ). qPCR analysis showed that expression of the mESC/epiblast markers Oct4 , Rex1 and Fgf5 was comparable between TSA and DMSO treatment at day 6; however, the expression of the NPC markers Sox1 , Pax6 and Sox3 decreased significantly with TSA treatment ( Fig. 2c ). In contrast, the expression of the mesoderm markers Mixl1 , T and Meox1 , as well as the definitive endoderm markers Foxa2 , Sox17 and Gata6 increased with TSA treatment ( Fig. 2c ). The decrease in the number of Sox1–GFP + or Pax6 + NPCs and the increase in the number of Flk1 + mesoderm cells or Gata6 + endoderm cells were further confirmed by immunocytochemical assays ( Fig. 2d,e ). Similar to TSA, two other HDACis, NaB and VPA, also reduced the percentages of GFP + NPCs in a dose-dependent manner ( Supplementary Fig. 2A ). In addition to the repression of neural differentiation in the monolayer culture, TSA treatment inhibited mESC neural differentiation in the embryonic body cultures ( Supplementary Fig. 2B,C ). Thus, these results suggest that HDACi such as TSA inhibits mESC neural fate commitment and promotes mesendoderm differentiation. 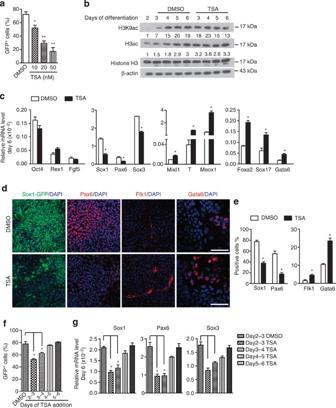Figure 2: HDACi inhibits mESC neural commitment and promotes mesendoderm differentiation. (a) Statistical analysis of Sox1–GFP+cells at day 6 (n=4). Day 2 cells were treated with DMSO or TSA (10 nM, 20 nM, 50 nM) for 24 h. (b) Western blotting analysis of H3ac and H3K9ac levels during mESC neural differentiation. Day 2 cells were treated with DMSO or TSA for 24 h, then removed and harvested from day 2 to day 6. (c) Gene expression analysis of day 6 cells described inb. Relative expression level was normalized bygapdh. (d) Sox1–GFP+, Pax6, Flk1 and Gata6 immunocytochemistry of the day 6 cells described inb. Scale bar, 75 μm. (e) Statistical analysis of Sox1+, Pax6+, Flk1+and Gata6+cells ind(n=4). (f) Statistical analysis of Sox1–GFP+cells at day 6 (n=4). DMSO or TSA was added at different time point from day 2 to day 5 for 24 h. (g) Gene expression analysis of day 6 cells described inf. Relative expression level was normalized bygapdh. Unless indicated, the data were shown from at least three independent experiments. Data inc,e–grepresent mean±s.d. *P<0.05, **P<0.01, Student’st-test. Figure 2: HDACi inhibits mESC neural commitment and promotes mesendoderm differentiation. ( a ) Statistical analysis of Sox1–GFP + cells at day 6 ( n =4). Day 2 cells were treated with DMSO or TSA (10 nM, 20 nM, 50 nM) for 24 h. ( b ) Western blotting analysis of H3ac and H3K9ac levels during mESC neural differentiation. Day 2 cells were treated with DMSO or TSA for 24 h, then removed and harvested from day 2 to day 6. ( c ) Gene expression analysis of day 6 cells described in b . Relative expression level was normalized by gapdh . ( d ) Sox1–GFP + , Pax6, Flk1 and Gata6 immunocytochemistry of the day 6 cells described in b . Scale bar, 75 μm. ( e ) Statistical analysis of Sox1 + , Pax6 + , Flk1 + and Gata6 + cells in d ( n =4). ( f ) Statistical analysis of Sox1–GFP + cells at day 6 ( n =4). DMSO or TSA was added at different time point from day 2 to day 5 for 24 h. ( g ) Gene expression analysis of day 6 cells described in f . Relative expression level was normalized by gapdh . Unless indicated, the data were shown from at least three independent experiments. Data in c , e – g represent mean±s.d. * P <0.05, ** P <0.01, Student’s t -test. Full size image To test whether the repression of neural differentiation by TSA was stage specific, TSA was added at different time points from day 2 to day 5 for 24 h, and NPC marker expression was measured at day 6. Compared with the control DMSO treatment, the percentages of Sox1–GFP + NPCs at day 6 as well as the expression of the NPC markers Sox1, Pax6 and Sox3 were reduced significantly with TSA treatment at day 2 and 3, the epiblast-like stage, but not at day 4 and 5, the NPCs stage ( Fig. 2f,g ). These results indicate that the cells at the epiblast-like stage are sensitive to TSA treatment. In addition, TSA treatment efficiently inhibited the neural differentiation of an EpiSC line derived from mouse embryos at E6.5 ( Supplementary Fig. 3A ). As expected, NaB treatment at the epiblast-like stage but not at the NPCs stage also resulted in the inhibition of mESC neural differentiation ( Supplementary Fig. 3B ). Together, all these observations suggest that histone deacetylation at the epiblast-like stage is essential for mESC neural fate commitment. HDAC1 plays a critical role in neural fate commitment To determine which HDACs are involved in the deacetylation during neural fate determination, qPCR was conducted to assess the expression of all 11 HDACs. qPCR data showed that compared with other HDACs including HDAC2 , HDAC3 , HDAC5 and HDAC6 , the expression of HDAC1 transcripts was most abundant in mESCs, epiblast-like cells at day 2 and NPCs at day 6 in vitro , as well as in E7.0 mouse embryos in vivo ( Fig. 3a , Supplementary Fig. 4A ). Western blotting confirmed that the expression of HDAC1 protein was maintained at high levels throughout mESC neural differentiation ( Fig. 3b ). 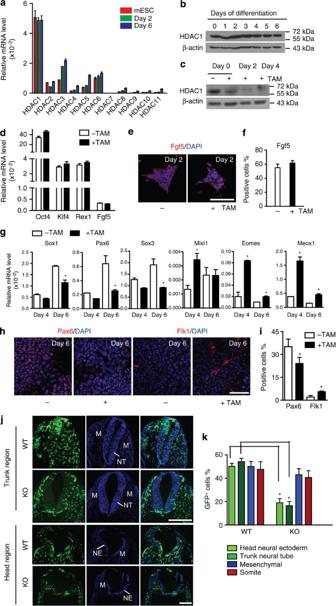Figure 3: Deletion ofHDAC1partially phenocopies defective mESC neural commitment by HDACi treatment. (a) Expression analysis of 11 histone deacetylases during mESC neural differentiation. Relative expression level was normalized bygapdh. (b) Western blotting analysis of the HDAC1 level during mESC neural differentiation. (c) Western blotting analysis of the HDAC1 level in cells treated with or without TAM. Cells were treated TAM (1 μM) at day 0, then harvested from day 0 to day 4. (d) Gene expression analysis of mESCs and the day 2 cells described inc. Relative expression level was normalized bygapdh. (e) Immunocytochemistry for Fgf5 in the day 2 cells described inc. Scale bar, 75 μm. (f) Statistical analysis of Fgf5+cells ine. (g) Gene expression analysis of day 4 and day 6 cells treated with or without TAM. Relative expression level was normalized bygapdh. (h) Immunocytochemistry for Pax6 and Flk1 in the day 6 cells described inc. Scale bar, 75 μm. (i) Statistical analysis of Pax6+and Flk1+cells inh(n=3). (j) Contribution of injected GFP+WT (HDAC1lox/lox) orHDAC1KO (HDAC1Δ/Δ) mESCs to different germ layers in E8.5–E9.0 chimeric embryos. Scale bar, 200 μm. (k) Statistical analysis of GFP+cell distribution in the various germ layer lineages described inj(WT,n=10; KO,n=6). Representative data of qPCR (a,d,g) were shown from three independent experiments. Data ina,d,f,g,i,krepresent mean±s.d. *P<0.05, Student’st-test. NE, neuroectoderm; NT, neural tube; M, mesenchyme. Figure 3: Deletion of HDAC1 partially phenocopies defective mESC neural commitment by HDACi treatment. ( a ) Expression analysis of 11 histone deacetylases during mESC neural differentiation. Relative expression level was normalized by gapdh . ( b ) Western blotting analysis of the HDAC1 level during mESC neural differentiation. ( c ) Western blotting analysis of the HDAC1 level in cells treated with or without TAM. Cells were treated TAM (1 μM) at day 0, then harvested from day 0 to day 4. ( d ) Gene expression analysis of mESCs and the day 2 cells described in c . Relative expression level was normalized by gapdh . ( e ) Immunocytochemistry for Fgf5 in the day 2 cells described in c . Scale bar, 75 μm. ( f ) Statistical analysis of Fgf5 + cells in e . ( g ) Gene expression analysis of day 4 and day 6 cells treated with or without TAM. Relative expression level was normalized by gapdh . ( h ) Immunocytochemistry for Pax6 and Flk1 in the day 6 cells described in c . Scale bar, 75 μm. ( i ) Statistical analysis of Pax6 + and Flk1 + cells in h ( n =3). ( j ) Contribution of injected GFP + WT ( HDAC1 lox/lox ) or HDAC1 KO ( HDAC1 Δ/Δ ) mESCs to different germ layers in E8.5–E9.0 chimeric embryos. Scale bar, 200 μm. ( k ) Statistical analysis of GFP + cell distribution in the various germ layer lineages described in j (WT, n =10; KO, n =6). Representative data of qPCR ( a , d , g ) were shown from three independent experiments. Data in a , d , f , g , i , k represent mean±s.d. * P <0.05, Student’s t -test. NE, neuroectoderm; NT, neural tube; M, mesenchyme. Full size image It has been reported that HDAC1 knockout led to embryonic lethality with compromised head formation at E9.5 (ref. 32 ). To investigate the function of HDAC1 in mESC neural fate determination, a conditional knockout mESC line ( HDAC1 lox/lox , Rosa26Cre-ER ) was used in the study [44] . The deletion of the HDAC1 gene was achieved by tamoxifen (TAM) treatment 2 days before mESC neural differentiation ( Fig. 3c ). The expression of Oct4 , Klf4 and Rex1 at day 0 and Fgf5 at day 2, as well as the number of Fgf5 + epiblast-like cells at day 2 was comparable with or without the TAM treatment ( Fig. 3d–f ). However, the expression of the NPC markers Sox1 , Pax6 and Sox3 at day 6 significantly decreased due to the HDAC1 depletion ( Fig. 3g ). In contrast, the expression of the mesendoderm markers Mixl1, Eomes and Meox1 significantly increased at day 4 or day 6 ( Fig. 3g ). Consistently, the percentage of Pax6 + NPCs decreased, while the number of Flk1 + mesoderm cells increased at day 6 with HDAC1 deficiency ( Fig. 3h,i ). These data indicate that HDAC1 is crucial for the appropriate mESC neural differentiation. Next, we asked whether HDAC1 participates in mESC neural fate commitment at the epiblast-like stage. mESC-derived EpiSCs (ESD-EpiSCs) were established from differentiated HDAC1 lox/lox , Rosa26Cre-ER mESCs at day 2 (see methods for details) [42] . The ESD-EpiSCs were pretreated with TAM before neural differentiation assays. As expected, HDAC1 deficiency resulted in the inhibition of neural fate and the promotion of the mesendoderm lineage in these ESD-EpiSCs ( Supplementary Fig. 4B ). Nevertheless, HDAC1 overexpression in the differentiated mESCs at the epiblast-like stage had little effect on the neural differentiation process, indicating that probably ectopic HDAC1 could not contribute further to the deacetylating activities conducted by the abundant endogenous HDACs ( Supplementary Fig. 4C–E ). Together, these data suggest that HDAC1 is required for mESC neural fate commitment especially at the transition from EpiSCs to NPCs. We further asked whether HDAC1 is imperative for the early neural development in vivo through chimeric mouse assays. To this, GFP-labelled wild-type (WT) or HDAC1 knockout (KO) mESCs were injected into the blastocyst, and embryos were transferred into pseudopregnant mice (see methods for details) [45] . Chimeric embryos were collected at E8.5–E9.0, and the contribution of GFP + cells was quantified in the chimeras generated from WT or HDAC1 KO mESCs, respectively. WT GFP + mESCs contributed equally to different cell lineages including neural tissues, mesenchyme and somite. By contrast, compared with that of the control, the incorporating rate of GFP + HDAC1 KO mESCs into the head neural ectoderm and trunk neural tube was significantly reduced ( Fig. 3j,k ). Clearly, HDAC1 is required for neural fate commitment in vivo . To determine the functions of other HDAC genes with relatively lower expression level, such as HDAC 2, HDAC 3, HDAC5 and HDAC6 , we used HDAC2 lox/lox , Rosa26Cre-ER mESCs to study the function of HDAC2 (ref. 44 ), and found that HDAC2 deficiency did not affect the neural differentiation of mESCs ( Supplementary Fig. 5A,B ). Similar to HDAC1 , knockdown of either HDAC5 or HDAC6 also inhibited 46C mESC neural differentiation ( Supplementary Fig. 5C–E ). In contrast, knockdown of HDAC3 promoted the neural differentiation of 46C mESCs ( Supplementary Fig. 5C–E ). Together, these results suggest that several HDACs participate in the regulation of mESC neural differentiation, and most likely, HDAC1 is one abundant deacetylase to ensure neural fate commitment. Identification of Nodal as a target of histone deacetylation To investigate the regulatory mechanisms of HDACi at the genome-wide level, complementary DNA microarrays were performed with the RNAs prepared from the differentiated cells at day 3 with or without 24 h TSA treatment initiated at day 2 (DMSO versus TSA). Differential gene expression analysis found that 873 genes showed more than twofold changes in expression; including 621 upregulated genes shown in the heat map ( Fig. 4a ). Gene ontology (GO) analysis revealed that the upregulated gene sets were highly enriched for biological functions related to mesoderm development, mesoderm morphogenesis and others ( Fig. 4b ). Detailed analysis showed that the mesoderm formation-related genes, such as the T-box genes Tbx6 and T , the homeobox genes Mixl1 and Evx1 , the bHLH gene Mesp1 and the morphogenetic genes Nodal , Wnt3a and Fgf8 were markedly upregulated by TSA treatment ( Fig. 4c ). The enhanced expression of these genes by TSA was further validated by qPCR ( Supplementary Fig. 6A ). These results indicate that the non-neural lineage genes, which are essential for mesoderm development, are repressed during mESC neural fate commitment but are ectopically activated by HDACi treatment. 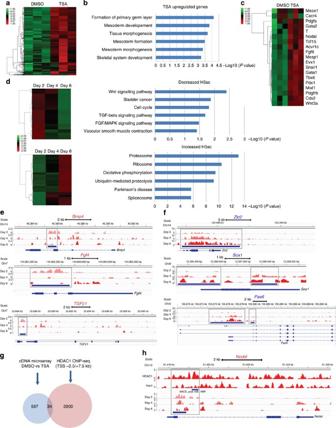Figure 4: Identification ofNodalas the deregulated target of histone deacetylation. (a) Hierarchical clustering of gene expression in the day 3 cells treated with DMSO or TSA (n=3). The colours indicate gene expression normalized in units of s.d. from the mean across samples (red, upregulation; green, downregulation). (b) GO analysis of TSA-upregulated genes. (c) Heat map showing TSA-upregulated genes involved in mesendoderm development. (d) KEGG pathways of genes with decreased or increased H3ac deposition in day 2, day 4 and day 6 cells. (e) Typical examples of decreased H3ac distribution in day 2, 4 and 6 cells. Peak calling was conducted based on MACS software, and the grey boxes represent the peak regions. (f) Typical examples of increased H3ac distribution in day 2, 4 and 6 cells. Peak calling was conducted based on MACS software, and the grey boxes represent the peak regions. (g) Venn diagram showing the overlap of upregulated genes by TSA and HDAC1 ChIP-seq target genes. (h) HDAC1 binding sites and the H3ac distribution at theNodallocus in day 2, 4 and 6 cells. Peak calling was conducted based on the MACS software, and the HDAC1 binding region is chr10_61419161_61419487. Figure 4: Identification of Nodal as the deregulated target of histone deacetylation. ( a ) Hierarchical clustering of gene expression in the day 3 cells treated with DMSO or TSA ( n =3). The colours indicate gene expression normalized in units of s.d. from the mean across samples (red, upregulation; green, downregulation). ( b ) GO analysis of TSA-upregulated genes. ( c ) Heat map showing TSA-upregulated genes involved in mesendoderm development. ( d ) KEGG pathways of genes with decreased or increased H3ac deposition in day 2, day 4 and day 6 cells. ( e ) Typical examples of decreased H3ac distribution in day 2, 4 and 6 cells. Peak calling was conducted based on MACS software, and the grey boxes represent the peak regions. ( f ) Typical examples of increased H3ac distribution in day 2, 4 and 6 cells. Peak calling was conducted based on MACS software, and the grey boxes represent the peak regions. ( g ) Venn diagram showing the overlap of upregulated genes by TSA and HDAC1 ChIP-seq target genes. ( h ) HDAC1 binding sites and the H3ac distribution at the Nodal locus in day 2, 4 and 6 cells. Peak calling was conducted based on the MACS software, and the HDAC1 binding region is chr10_61419161_61419487. Full size image Next, we asked how histone acetylation/deacetylation modifications participate in the regulation of neural differentiation. To identify potential target genes regulated by histone acetylation at the global level, H3ac chromatin immunoprecipitation (ChIP)-seq assays were performed with chromatin prepared from the differentiated cells at day 2, 4 and 6, respectively. Through model-based analysis (MACS) [46] , we found numerous genomic loci with either upregulated or downregulated H3ac modifications. Among the gene sets, genomic loci of which showed progressive and significant decrease of H3ac levels, three signalling pathways, TGF-beta, FGF/MAPK and WNT were identified by GO enrichment analysis ( Fig. 4d ). These pathways have been shown to negatively regulate neural fate determination [1] , [4] , [47] . Indeed, detailed analysis revealed that the enrichment of H3ac was gradually decreased on the loci of Bmp4 , Fgf4 , TGFβ1 and Nodal genes, which play important roles in mouse and human ESC mesendoderm differentiation [48] , [49] , [50] ( Fig. 4e,h ). In addition, among the gene sets, genomic loci of which displayed increased H3ac levels, several functional pathways such as proteasome, ribosome and oxidative phosphorylation, were identified. Interestingly, the enrichment of H3ac was gradually elevated on the loci of neural genes, such as Zic2 , Sox1 and Pax6 ( Fig. 4f ). The observations above suggest that the global histone deacetylation is probably associated with the genes of neural inhibitory pathways (TGF-beta, FGF/MAPK and WNT) to repress their expression during mESC neural fate commitment. Since the loss of HDAC1 partially phenocopied the inhibitory effect of HDACi on mESC neural determination, the targets of HDAC1 may mediate the effect of TSA. Therefore, the genome-wide ChIP-seq assay was also conducted to determine possible HDAC1 target genes. To enhance the binding specificity and affinity for ChIP-seq, HDAC1 -rescued HDAC1 Δ/Δ+3 × Flag mESCs, in which a multiple epitope-tagged HDAC1 ( 3 × Flag-mHDAC1 ) was introduced into HDAC1 Δ/Δ mESCs were generated. The transcript and protein level of HDAC1 in HDAC1 Δ/Δ+3 × Flag mESCs were similar to that of endogenous HDAC1 in the control HDAC1 lox/lox mESCs ( Supplementary Fig. 6B,C ). qPCR showed that the expression of pluripotency genes ( Oct4 , Klf4 and Rex1 ) was not significantly altered in HDAC1 lox/lox , HDAC1 Δ/Δ and HDAC1 Δ/Δ+3 × Flag mESCs ( Supplementary Fig. 6D ). Next, ChIP-seq was conducted with a Flag tag antibody and chromatin prepared from differentiating day 2 cells of HDAC1 Δ/Δ+3 × Flag mESCs. About 2,834 binding peaks of HDAC1 were identified at the gene promoter regions from 2.5 kb upstream to 7.5 kb downstream of the transcription start site ( Supplementary Fig. 6E ). By integrating the HDAC1 ChIP-seq and microarray data, 34 genes, which were bound by HDAC1 and upregulated by TSA treatment, were identified ( Fig. 4g , Supplementary Table 1 ). ChIP–qPCR was performed to validate the binding of HDAC1 on genes such as Arg2 and Mesp1 , and qPCR was conducted to confirm the enhanced expression of genes such as Arg2 , Mesp1 , Zfpm1 , Cldn26 and Nrgn by TSA treatment ( Supplementary Fig. 6F,G ). Interestingly, the Nodal gene, which encodes a ligand of the TGF-beta signalling pathway, was one of 34 genes identified in the assays ( Supplementary Table 1 ). HDAC1 was enriched at a conserved region of Nodal gene, defined as HDAC1 binding region (HBR) ( Fig. 4h ). In addition, H3ac ChIP-seq data showed that H3ac was enriched at the HBR in day 2 cells as well, and the local H3ac levels were decreased gradually during the neural differentiation at day 4 and day 6 ( Fig. 4h ). Thus, these results suggest Nodal as one of the target genes that potentially mediates the neural inhibition of HDACi during mESC neural differentiation. Regulatory function of HBR in Nodal gene expression It has been well-known that Nodal signalling participates in neural and mesendoderm fate decision as an important mesendoderm-inducing morphogen during ESC differentiation [51] , [52] , [53] . We then asked the epigenetic mechanism underlying Nodal gene expression, potentially through histone deacetylation. We confirmed the binding of HDAC1 on HBR by ChIP–qPCR ( Fig. 5a ). Interestingly, the HBR is localized in a conserved regulatory asymmetric enhancer element that contains two FoxH1 binding sites [54] , [55] ( Supplementary Fig. 7A ). The enrichment of H3ac at the HBR was significantly enhanced by HDAC1 deficiency or TSA treatment ( Fig. 5b,c ). Furthermore, during mESC neural differentiation, both H3ac and H3K9ac levels at the HBR were relatively high at day 0 and day 2, then declined significantly at day 4 and day 6, indicating that the histone acetylation of HBR was dynamic ( Fig. 5d,e ). Consistently, binding of the phosphorylated polymerase II to Nodal gene promoter decreased on mESC neural differentiation ( Fig. 5f ), which correlated well with the reduced expression of Nodal transcripts and phosphorylated Smad2 protein (pSmad2, an indicator of Nodal signalling activity) ( Fig. 5g , Supplementary Fig. 7B ). 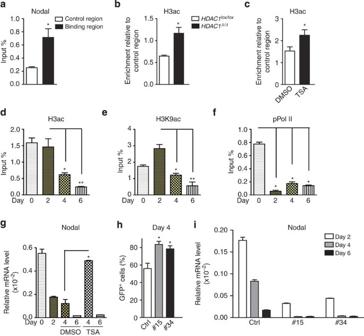Figure 5: Histone acetylation/deacetylation of HBR regulates the expression ofNodal. (a) ChIP–qPCR assay in day 2 cells. Enrichments of HDAC1 at the binding region (HBR) of theNodallocus were normalized with the control region (∼1 kb downstream of HBR region). (b) Analysis of H3ac levels on the HBR in day 4 cells differentiated from WT orHDAC1KO mESCs by H3ac ChIP–qPCR. (c) Analysis of H3ac levels on the HBR in day 3 cells treated with DMSO or TSA by H3ac ChIP–qPCR. (d) Analysis of H3ac levels on the HBR during mESC neural differentiation. (e) Analysis of H3K9ac levels on the HBR during mESC neural differentiation. (f) Analysis of phosphorylated RNA polymerase II (pPol II) binding on the promoter ofNodalduring mESC neural differentiation. (g) Expression analysis ofNodalduring mESC neural differentiation with DMSO or TSA treatment. Relative expression level was normalized bygapdh. (h) Statistical analysis of Sox1–GFP+cells at day 4. Cells were differentiated from control WT 46C or HBR-deleted 46C (#15 and #34). (i) Expression analysis ofNodalduring neural differentiation of control WT 46C or HBR-deleted 46C (#15 and #34). Relative expression level was normalized bygapdh. Representative data of ChIP–qPCR (a–f) and qPCR (g,i) were shown from three independent experiments. Data represent mean±s.d. *P<0.05, **P<0.01, Student’st-test. Figure 5: Histone acetylation/deacetylation of HBR regulates the expression of Nodal . ( a ) ChIP–qPCR assay in day 2 cells. Enrichments of HDAC1 at the binding region (HBR) of the Nodal locus were normalized with the control region ( ∼ 1 kb downstream of HBR region). ( b ) Analysis of H3ac levels on the HBR in day 4 cells differentiated from WT or HDAC1 KO mESCs by H3ac ChIP–qPCR. ( c ) Analysis of H3ac levels on the HBR in day 3 cells treated with DMSO or TSA by H3ac ChIP–qPCR. ( d ) Analysis of H3ac levels on the HBR during mESC neural differentiation. ( e ) Analysis of H3K9ac levels on the HBR during mESC neural differentiation. ( f ) Analysis of phosphorylated RNA polymerase II (pPol II) binding on the promoter of Nodal during mESC neural differentiation. ( g ) Expression analysis of Nodal during mESC neural differentiation with DMSO or TSA treatment. Relative expression level was normalized by gapdh . ( h ) Statistical analysis of Sox1–GFP + cells at day 4. Cells were differentiated from control WT 46C or HBR-deleted 46C (#15 and #34). ( i ) Expression analysis of Nodal during neural differentiation of control WT 46C or HBR-deleted 46C (#15 and #34). Relative expression level was normalized by gapdh . Representative data of ChIP–qPCR ( a – f ) and qPCR ( g , i ) were shown from three independent experiments. Data represent mean±s.d. * P <0.05, ** P <0.01, Student’s t -test. Full size image To further investigate the function of HBR in regulating Nodal gene expression, we utilized CRISPR (clustered regularly interspaced short palindromic repeats)–Cas9 system to delete the HBR of Nodal gene ( Supplementary Fig. 7A ). As previously reported [56] , [57] , the 46C mESCs were transiently transfected with plasmids containing mCherry, Cas9 and two sgRNAs targeting the genomic regions around HBR. Then, single cells were sorted to derive cell lines, and validated for the HBR deletion (see methods for details). Two clones with HBR deletion (#15 and #34) were chosen for the further study ( Supplementary Fig. 7C–E ). Interestingly, the percentages of GFP + NPCs in the HBR-deleted mESCs (#15 and #34) at differentiating day 4 were significantly higher than the control (46C-sgLacZ) mESCs, and the expression of Nodal was markedly decreased during the differentiation ( Fig. 5h,i ). In addition, the neural inhibitory effect of TSA was significantly relieved in the HBR-deleted mESCs ( Supplementary Fig. 7F ). Since the HBR was located within the asymmetric enhancer element that is essential for FoxH1 -regulated Nodal expression in vivo , the decreased Nodal expression on HBR deletion in mESCs could be due to loss of positive regulation by essential transcription factors such as FoxH1. We found that the lack of FoxH1 resulted in the decreased expression of Nodal and the increased percentages of Sox1–GFP + NPCs during neural differentiation (data not shown). Thus, these results reveal that the conserved HBR serves as an elaborated element, which coordinates transcription factors and epigenetic modifications to regulate Nodal expression and neural fate determination. Nodal signalling inhibition partly mimics histone deacetylation Nodal expression was upregulated on HDACi treatment or loss of HDAC1 ; therefore, we asked whether Nodal signalling activity was also subsequently enhanced. Indeed, the pSmad2 level was increased when the cells were treated with TSA for 24 h at day 2 ( Fig. 6a ). Next, we asked whether the inhibition of Nodal signalling activity affected neural repression mediated by TSA treatment. Either SB431542 (SB), a Nodal signalling inhibitor, or Noggin, a BMP antagonist, was added at day 2 during mESC neural differentiation. SB but not Noggin rescued the neural inhibition of TSA ( Fig. 6b,c , Supplementary Fig. 8A–C ). Consistently, knockdown of Nodal gene also promoted mESC neural differentiation, which was not affected by the TSA treatment ( Fig. 6d , Supplementary Fig. 8D,E ). These results suggest that Nodal signalling may be one of the major pathways mediating TSA inhibition on mESC neural fate determination. To further validate this notion, day 2 cells were treated with activin, a Nodal agonist, together with TSA. Dual treatments repressed mESC neural conversion synergistically ( Fig. 6e ). To investigate whether Nodal also mediates the mesendoderm-promoting activity of TSA, mESC was induced to mesendoderm differentiation in chemically defined medium as previously described [58] . As expected, the percentage of Cxcr4 + mesendoderm cells increased by TSA treatment, which was repressed by SB treatment ( Supplementary Fig. 9A ). In contrast, the treatment of both activin and TSA further enhanced the mESC mesendoderm differentiation ( Supplementary Fig. 9A,B ). These data indicate that TSA inhibits mESC neural determination and promotes mesendoderm differentiation at least partially by activating the Nodal signalling pathway. 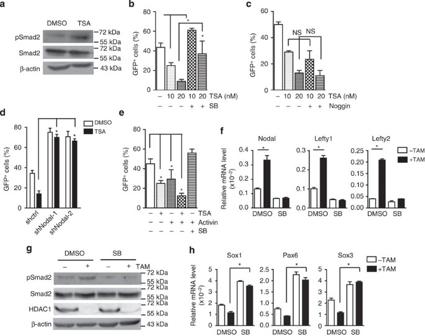Figure 6: The inhibition of Nodal signalling rescues mESC neural fate repression by TSA treatment orHDAC1deletion. (a) Western blotting analysis of pSmad2 in the day 3 cells treated with DMSO or TSA at day 2 for 24 h. (b) Statistical analysis of Sox1–GFP+cells at day 4 (n=3). The day 2 cells were treated with DMSO, TSA (10 nM, 20 nM) or TSA+SB (2 μM) for 24 h. (c) Statistical analysis of Sox1–GFP+cells at day 4 (n=3). The day 2 cells were treated with DMSO, TSA (10 nM, 20 nM) or TSA+Noggin (100 ng ml−1) for 24 h. (d) Statistical analysis of Sox1–GFP+cells at day 4 (n=4). Control-mESCs (shctrl) andNodalknockdown-mESCs (shNodal-1 and shNodal-2) were treated with DMSO or TSA for 24 h at day 2. (e) Statistical analysis of Sox1–GFP+cells at day 4 (n=4). The day 2 cells were treated with DMSO, TSA (10 nM), activin (1 ng ml−1), TSA+activin or activin+SB (2 μM) for 24 h. (f) Gene expression analysis of the Nodal signalling target genes in the day 4 cells differentiated fromHDAC1lox/loxmESCs. DMSO or SB was added at day 2 for 24 h, and TAM was added in the stock culture before differentiation. Relative expression level was normalized bygapdh. (g) Western blotting analysis of pSmad2. DMSO or SB (20 μM) was added at day 2 for 24 h, and TAM was added in the stock culture before differentiation. (h) Gene expression analysis of the NPC markers at day 6. DMSO or SB (20 μM) was added at day 2, and TAM was added in the stock culture before differentiation. Relative expression level was normalized bygapdh. Representative data of qPCR (f,h) were shown from at least three independent experiments. Data inb–f,hrepresent mean±s.d. *P<0.05, Student’st-test. NS, not significant. Figure 6: The inhibition of Nodal signalling rescues mESC neural fate repression by TSA treatment or HDAC1 deletion. ( a ) Western blotting analysis of pSmad2 in the day 3 cells treated with DMSO or TSA at day 2 for 24 h. ( b ) Statistical analysis of Sox1–GFP + cells at day 4 ( n =3). The day 2 cells were treated with DMSO, TSA (10 nM, 20 nM) or TSA+SB (2 μM) for 24 h. ( c ) Statistical analysis of Sox1–GFP + cells at day 4 ( n =3). The day 2 cells were treated with DMSO, TSA (10 nM, 20 nM) or TSA+Noggin (100 ng ml −1 ) for 24 h. ( d ) Statistical analysis of Sox1–GFP + cells at day 4 ( n =4). Control-mESCs (shctrl) and Nodal knockdown-mESCs (shNodal-1 and shNodal-2) were treated with DMSO or TSA for 24 h at day 2. ( e ) Statistical analysis of Sox1–GFP + cells at day 4 ( n =4). The day 2 cells were treated with DMSO, TSA (10 nM), activin (1 ng ml −1 ), TSA+activin or activin+SB (2 μM) for 24 h. ( f ) Gene expression analysis of the Nodal signalling target genes in the day 4 cells differentiated from HDAC1 lox/lox mESCs. DMSO or SB was added at day 2 for 24 h, and TAM was added in the stock culture before differentiation. Relative expression level was normalized by gapdh . ( g ) Western blotting analysis of pSmad2. DMSO or SB (20 μM) was added at day 2 for 24 h, and TAM was added in the stock culture before differentiation. ( h ) Gene expression analysis of the NPC markers at day 6. DMSO or SB (20 μM) was added at day 2, and TAM was added in the stock culture before differentiation. Relative expression level was normalized by gapdh . Representative data of qPCR ( f , h ) were shown from at least three independent experiments. Data in b – f , h represent mean±s.d. * P <0.05, Student’s t -test. NS, not significant. Full size image In HDAC1 lox/lox , Rosa26Cre-ER mESCs, the expression of Nodal and its downstream targets, Lefty1 and Lefty2 , was increased by TAM-induced HDAC1 deletion, and SB treatment abolished this upregulation ( Fig. 6f ). Similarly, western blotting analysis revealed that the pSmad2 level was increased in differentiated HDAC1 Δ/Δ mESCs at day 3, which was also reversed by SB treatment ( Fig. 6g ). Then, we asked whether SB rescues the inhibitory effect on neural differentiation by HDAC1 deficiency. Addition of SB partially recovered the decreased expression of the NPC markers Sox1 , Pax6 and Sox3 in differentiated HDAC1 Δ/Δ mESCs at day 6 ( Fig. 6h ). In contrast, the mesendoderm-promoting effect of HDAC1 deletion was inhibited by SB treatment ( Supplementary Fig. 9C ). Together, these results suggest that the activation of Nodal signalling partially mediates the neural inhibition and mesendoderm promotion activities of HDACi treatment or HDAC1 loss. Histone deacetylation ensures neural fate commitment ex vivo The anterior epiblast in mouse embryos at E7.0 gives rise to the neuroectodermal layer; meanwhile, the posterior epiblast generates the mesoderm and the endoderm [59] . Our observations above demonstrated that histone deacetylation regulates the fate choice between the neural and mesendoderm lineages by modulating the Nodal pathway in pluripotent stem cells in vitro ; therefore, we asked whether this regulation is also conserved in early mouse embryos in vivo . To answer the question, E7.0 mouse embryos were collected [60] , and immunocytochemistry assays were performed on series of transverse sections from the distal to the proximal planes with a specific antibody against H3ac. As expected, the heterogeneous distribution of H3ac was observed at the proximal plane but not at the middle and distal planes. The H3ac level in the anterior proximal cells with prospective neuroectoderm fate was significantly lower than in the posterior proximal region where the mesendoderm progenitor is localized ( Fig. 7a,b ), suggesting that the lower H3ac level in the anterior proximal region may be necessary for neural fate commitment during early mouse development in vivo . 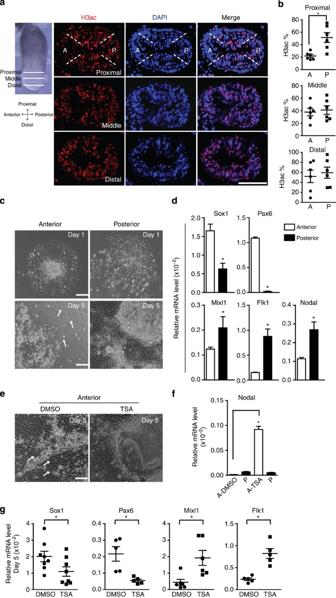Figure 7: TSA treatment represses neural fate commitment of the anterior epiblast at E7.0. (a) Immunocytochemistry for H3ac in E7.0 mouse embryos. Transverse sections from distal to proximal were shown. Scale bar, 75 μm. (b) Statistical analysis of H3ac+cells ina(n=6). (c) Representative cellular morphologies of day 1 and day 5 cells differentiated in N2B27 medium from the anterior and posterior explants. The images were shown representatively for one of the three biological repeats. The arrows show the neurite outgrowth. Scale bar, 200 μm. (d) Gene expression analysis of the day 5 cells. Relative expression level was normalized bygapdh. (e) Representative cellular morphologies of the day 5 cells differentiated from the anterior explants with DMSO or TSA treatment. The images were shown representatively for one of three biological repeats. The arrows show the neural cell-specific neurite outgrowth. Scale bar, 200 μm. (f) Gene expression analysis ofNodal. After attachment at day 1, the anterior cells were treated with DMSO (A-DMSO) or TSA (A-TSA) for 24 h, and harvested for the messenger RNA expression analysis. Relative expression level was normalized bygapdh. (g) Gene expression analysis of the day 5 cells described ine. (Sox1,n=8; Pax6,n=5; Mixl1,n=6; Flk1,n=5). Relative expression level was normalized bygapdh. Representative data of qPCR (d,f) were shown from three independent experiments. Data inb,d,f,grepresent mean±s.d. *P<0.05, Student’sttest. Figure 7: TSA treatment represses neural fate commitment of the anterior epiblast at E7.0. ( a ) Immunocytochemistry for H3ac in E7.0 mouse embryos. Transverse sections from distal to proximal were shown. Scale bar, 75 μm. ( b ) Statistical analysis of H3ac + cells in a ( n =6). ( c ) Representative cellular morphologies of day 1 and day 5 cells differentiated in N2B27 medium from the anterior and posterior explants. The images were shown representatively for one of the three biological repeats. The arrows show the neurite outgrowth. Scale bar, 200 μm. ( d ) Gene expression analysis of the day 5 cells. Relative expression level was normalized by gapdh . ( e ) Representative cellular morphologies of the day 5 cells differentiated from the anterior explants with DMSO or TSA treatment. The images were shown representatively for one of three biological repeats. The arrows show the neural cell-specific neurite outgrowth. Scale bar, 200 μm. ( f ) Gene expression analysis of Nodal . After attachment at day 1, the anterior cells were treated with DMSO (A-DMSO) or TSA (A-TSA) for 24 h, and harvested for the messenger RNA expression analysis. Relative expression level was normalized by gapdh . ( g ) Gene expression analysis of the day 5 cells described in e . (Sox1, n =8; Pax6, n =5; Mixl1, n =6; Flk1, n =5). Relative expression level was normalized by gapdh . Representative data of qPCR ( d , f ) were shown from three independent experiments. Data in b , d , f , g represent mean±s.d. * P <0.05, Student’s t test. Full size image To test this hypothesis, the extra embryonic endoderm (ExE) and visceral endoderm were carefully removed from E7.0 mouse embryos, the epiblast was dissected into the anterior (A) and posterior (P) region, then we cultured the tissues in serum-free medium for 5 days as previously described [61] . After the tissue explants attached for 1 day, the anterior parts displayed homogenous epiblast-like cells with a high nuclear-cytoplasmic ratio; however, the posterior parts generated compact epithelial cells in the centre surrounded by scattered migrating mesoderm-like cells ( Fig. 7c , upper panel). On day 5, the cells of the anterior regions generated long neurite-like projections ( Fig. 7c , lower panel, arrows) and expressed higher levels of the NPC markers Sox1 and Pax6 ( Fig. 7d ). The cells from the posterior explants primarily differentiated into beating cardiac muscle cells and expressed high levels of mesodermal markers such as Mixl1, Flk1 and Nodal ( Fig. 7c,d ). We asked whether histone deacetylation regulates the cell fate of the anterior epiblast. The attached anterior explants were treated with DMSO or TSA for 24 h and cultured for 3 more days. At day 5, the TSA-treated anterior tissues showed much less neurite-like projections compared with the DMSO-treated control tissues ( Fig. 7e ). Consistently, the expression of Nodal in the anterior explants was significantly upregulated after TSA treatment ( Fig. 7f ). Intriguingly, in the anterior explants treated with TSA, the expression of the NPC markers Sox1 and Pax6 was reduced; nonetheless, the expression of the posterior mesoderm markers Mixl1 and Flk1 was significantly increased ( Fig. 7g ). Together, these results indicate that the histone deacetylation event occurring in the anterior proximal region of the mouse embryo may restrict the expression of Nodal to ensure neuroectoderm development and to prevent the mesendoderm development. In this study, we find that histone deacetylation occurs at the epiblast-like stage and correlates with neural fate determination during mESC neural differentiation. We show that inhibition of histone deacetylation by either HDACi or loss of HDAC1 gene inhibits neural fate commitment while promotes mesendoderm fate in vitro and ex vivo . We further identify Nodal as a major target to mediate the effects of HDACi or HDAC1 deficiency. Thus, histone deacetylation, as an important epigenetic modification, can actively participate in the early neural fate commitment by repressing Nodal signalling. Neural fate determination is accomplished by the coordination between the inhibition of the extrinsic posterior signals and the activation of intrinsic factors. However, whether and how epigenetic regulations participate in early neural induction remains largely unknown. The lower level of H3ac is observed at the epiblast-like stage of mESC neural differentiation in vitro and in the anterior proximal region of mouse embryos at E7.0 in vivo . Our previous studies revealed that cell populations in the anterior proximal region of mouse embryos at E7.0 possess bipotentiality to form either the surface or the neural ectoderm depending on the local cues [61] . These observations indicate that the transient histone deacetylation most likely participates in the neural fate commitment. The involvement of HDAC1 and HDAC2 in late neurogenesis of mouse brain development has been well-studied [33] , [34] . Nonetheless, how HDAC1 participates in the early neural commitment hasn’t been elucidated. Consistent with previous observations in mouse embryos [32] , neural differentiation is also impaired in HDAC1 -deficient mESCs in vitro , which partially phenocopies HDACi treatment. In addition, chimeric assays reveal the markedly reduced contribution of HDAC1 -deficient mESCs to neural tissues in early mouse embryos as compared with the WT mESCs. Moreover, the neural development of the anterior explants of mouse embryos is compromised in the presence of TSA. Therefore, these results suggest that transient histone deacetylation involving HDAC1 at the epiblast phase plays a critical role in the murine neural fate commitment. In addition to HDAC1, knockdown of HDAC5 or HDAC6 results in impaired mESC neural differentiation as well. Conversely, knockdown of HDAC3 promotes mESC neural differentiation, which is consistent with the observation of neural differentiation in human ESCs [62] , [63] . Therefore, HDACs might orchestrate with each other to ensure mESC neural fate commitment. Mechanistically, we have identified Nodal gene, encoding the ligand of Nodal signalling, as a target regulated by histone deacetylation. As an important morphogen involved in the establishment of the A–P axis, the specific repression of Nodal signalling by its antagonists, Cer1 and Lefty1 (secreted from anterior visceral endoderm cells), is crucial for neural fate commitment and the appropriate patterning of the primitive streak [1] , [3] . However, other than the extrinsic Nodal signalling antagonists, little is known about the intrinsic mechanisms underlying Nodal expression in the anterior epiblast cells. We have found that both HDAC1 and H3ac are enriched at the conserved HBR of Nodal gene, and H3ac levels are dynamic following the neural differentiation. Moreover, either HBR deletion or downregulation of FoxH1 leads to decreased Nodal expression, as well as enhanced neural differentiation. Most likely, the histone acetylation at the HBR may result in chromatin remodelling, which allows for the access of transcriptional factors such as FoxH1 to activate Nodal expression. Here we would like to propose an intrinsic mechanism that histone deacetylation at the conserved HBR is a repressive epigenetic modification to limit Nodal gene expression, which ensures mESC neural fate determination. However, we can’t exclude that other unknown regulatory machineries could also participate in the regulation of Nodal expression. During gastrulation, the cell lineage specification is tempo-spatially controlled by extracellular signals and intracellular transcription factors. Here we find that in the prospective neuroectoderm of the early mouse embryos, transient histone deacetylation is also an imperative epigenetic modification, and it is a key intracellular event to limit the expression of Nodal, and to ensure the appropriate neural initiation. Thus, our study would provide new insight on how intrinsic programmes mediated by the epigenetic factors such as HDACs participate in the neural fate commitment. Cell culture and differentiation mESC lines E14tg2a, 46C, HDAC1 lox/lox , Rosa26Cre-ER mESC and HDAC2 lox/lox , Rosa26Cre-ER mESC were used in this study and cultured in feeder-free medium [64] . Monolayer culture for neural differentiation was performed as previously described [40] . Briefly, ESCs were plated onto 0.1% gelatin-coated dishes and cultured in N2B27 medium at the density of 0.5–1 × 10 4 cm −2 . N2B27 medium comprises 50% DMEM/F12 and 50% Neurobasal medium (both from GIBCO) supplemented with 1 × N2, 1 × B27 (GIBCO), 0.1% bovine serum albumin fraction V (Roche), 1 mM Glutamine (GIBCO) and 0.1 mM β-mercaptoethanol (GIBCO). For neural differentiation in suspension [41] , dissociated ESCs were suspended in the Petri dish and cultured in GMEM (GIBCO) supplemented with 8% knockout serum replacement (GIBCO), 1 mM Glutamine, 1 mM pyruvate, 0.1 mM nonessential amino acids and 0.1 mM β-mercaptoethanol (all from GIBCO). To derive HDAC1 lox/lox ESD-EpiSCs, day 2 cells differentiated from HDAC1 lox/lox mESCs were dissociated into single cells and seeded in N2B27 medium supplemented with 20 ng ml −1 activin (R&D Systems) and 12 ng ml −1 bFGF (Invitrogen). Dishes should be coated with FBS for 24 h and washed with PBS before use. After 6 days, the surviving cells formed colonies. The colonies were picked, passaged every 2 days using collagenase IV (Invitrogen) and the medium was changed every day [42] . RNA preparation and qPCR analysis Total RNA was extracted from cells using Trizol reagent (Shanghai Pufei Biotechnology). About 1 μg total RNA was reversed and qPCR was performed using an Eppendorf Realplex2 (ref. 65 ). The primers used are listed in Supplementary Table 2 . Immunocytochemistry Cells were fixed in 4% paraformaldehyde (PFA) for 20 min at room temperature, blocked and stained with primary antibodies at 4 °C overnight [66] . For mouse embryos, according to the PS morphology, ICR embryos with decidua in proper stage were collected and fixed in 4% PFA at 4 °C for 1 h, then dehydrated in 20–30% sucrose overnight at 4 °C. Transverse 10 μm sections were taken using Leica CM 1950. After antigen retrieval with microwave in target retrieval solution (Dako) and 3% H 2 O 2 treatment, sections were blocked and stained with antibodies. The following primary antibodies were used: anti H3ac (1:200; Millipore 06–599), anti Tuj1 (1:500; Sigma), anti Pax6 (1:300; Convance), anti Flk1 (1:100; R&D Systems), anti Gata6 (10 μg ml −1 ; R&D Systems). Microarray analysis Total RNA was extracted, labelled and hybridized to Agilent Whole Mouse Genome Oligo 4 × 44 K Microarrays (one-colour platform) according to the manufacturer’s protocols. The comparison of day 3 cells treated with DMSO or TSA for 24 h was carried out with three biological replicates. For Agilent array data, we used limma package in R to get the expression of each probe. ‘Normexp’ was used for background normalization and ‘quantile’ for normalization between arrays. We calculated expression of each gene based on the average of probes and used Rankprod package in R to get the upregulated and downregulated genes with P value <0.005 as a cutoff. ChIP-sequence and data analysis Cells were cross-linked, lysed and sonicated to generate DNA fragments with an average size of 200 bp (ref. 67 ). About 10–15 ng IP DNA and input DNA measured by Qubit Fluorometer (Invitrogen) were used to construct DNA library by using ChIP-Seq Sample Prep Kit (Illumina). Enriched DNA sequencing was performed on Genome Analyzer IIx (Illumina). Reads were uniquely mapped to mm10 using bowtie (version 0.12.8), then peaks were called using MACS (macs 14 1.4.2) with default parameter. Genes with increased or decreased H3ac peaks were performed with GO enrichment analysis (DAVID). We defined genes bound by HDAC1 if peaks were identified by MACS at gene promoter region (upstream 2.5 kb and downstream 7.5 kb of transcription start site). The primers used are listed in Supplementary Table 3 . Mouse embryo explant culture Mouse ICR strain embryos with proper stage (E7.0) were collected from the decidua in DMEM/F12 medium containing 10% FBS (GIBCO). After removing the Reichert’s membrane and visceral endoderm cells with needles, embryo was cut off the ExE and separated into anterior and posterior parts to seed in the dish coated with FBS [61] . After attaching overnight in N2B27 medium, the anterior cells were treated with DMSO or TSA (10 nM) for 24 h, then removed and washed with PBS. After 3 days of spontaneous differentiation in N2B27 medium, cells were harvested and gene expression was analysed. Western blot Cells were lysed and subjected to Western blot analysis as described previously [68] . The following primary antibodies were used: HDAC1 (1:2,000; Millipore), Flag (1:2,000; Sigma), β-actin (1:10,000; Sigma), pSmad2 (1:1,000; Cell Signaling Technology), Smad2 (1:2,000; Cell Signaling Technology), Histone H3 (1:10,000; Sigma), H3ac (1:10,000; Millipore) and H3K9ac (1:1,000; Abcam). Original images of the Western blots can be found in Supplementary Fig. 10 . Flow cytometry analysis For the analysis of Sox1–GFP + percentages, cells were dissociated into single cells and analysed by FACS Calibur flow cytometer (Becton Dickinson, San Jose, CA). For the analysis of Cxcr4 + percentages, 1 × 10 5 cells were stained in 100 μl washing buffer with allophycocyanin (APC)-conjugated Cxcr4 antibodies at 4 °C for 30 min, followed by washing and analysis (17-9991-80, eBioscience). For cell apoptosis detection, day 4 cells were incubated with APC-labelled annexin V and manipulated as per the manufacturer’s instructions (88–8007, eBioscience). Isotope antibodies were used as negative controls. Data were analysed with FlowJo software (Tree Star, Ashland, OR). Gene knockdown and overexpression For gene knockdown in mESCs, the corresponding short hairpin RNAs (shRNAs) and control shRNA against Luciferase gene were cloned into the pLKO.1 constructs (Addgene). For the overexpression of HDAC1 , the complementary DNA was inserted into pCDH-EF1-Puro vector (Systems Biosciences), the production and infection of lentivirus supernatant was performed as described previously [45] . Briefly, after infection of lentivirus for 24 h, stable mESCs were selected by puromycin (2 μg ml −1 , Sigma). For HDAC3 , HDAC5 and HDAC6 knockdown during mESC differentiation, day 1 cells were infected with concentrated lentiviral particles for 6 h and washed with differentiation medium. The shRNA sequences are shown in Supplementary Table 4 . CRISPR/Cas9-mediated HBR deletion and validation in mESCs The control sgRNA-targeting LacZ (5′-CACCGTGCGAATACGCCCACGCGAT-3′) [57] , sgRNA-1 (Nodal-oligo1: 5′-CACCGCTCACCAGAGTAGGCCGAC-3′) and sgRNA-2 (Nodal-oligo2: 5′-CACCGCTGTCCGACCCTAGGCGGAG-3′) targeting the 5′ and 3′ regions of HBR were designed, annealed and ligated to the pX330 plasmid containing Cas9 and mCherry, respectively [69] . These pX330 plasmids were transfected into 46C mESCs using Lipofectamine 2,000 (Invitrogen) according to the manufacturer’s instructions. 24 h later, the single mCherry + cells were sorted and plated into 96-well plates individually through Aria II (Becton Dickinson). The 40 monoclones were randomly picked up and the genomic DNA of these clones was extracted for the validation of HBR deletion by regular PCR with primers spanning HBR (forward: 5′-GAACTCAGGCAACTCTCGTG-3′, reverse: 5′-TCAGGTGACTGCAAAACCGAA-3′). The deletion of HBR will produce a shorter band ( ∼ 340 bp), which was further validated by the DNA sequencing. Using the primers within HBR, we further performed qPCR to identify the clones with least ratio of HBR/control region, the nine clones and control WT clone were analysed, #15 and #34 with least ratio were used for further study. HBR: (Forward: 5′-AGTTCGGACTCAGGACTACCTTCC-3′, Reverse: 5′-AGACCGGATTAGAAGATGTGGATTGC-3′), Control region: (Forward: 5′-CCACCAGCACAGGCACCATCTA-3′, Reverse: 5′-AGTGAGTTCCAGGACAGCCAAGG-3′) Mouse chimeric embryos analysis Chimeric embryos analysis was performed as described previously [45] . Briefly, GFP-labelled WT mESCs ( HDAC1 lox/lox ) and HDAC1 KO mESCs ( HDAC1 Δ/Δ ) were injected into E2.5 mouse blastocysts, respectively, and then transferred into the uteri of day 2.5 pseudopregnant female mice. Chimeras at E8.5 to E9.0 were collected (WT, n =10; KO, n =6) and transverse sections were analysed to quantify the GFP-positive signals. Mouse care and treatment was approved by the Institutional Animal Care and Use Committee of the Shanghai Institutes for Biological Sciences, Chinese Academy of Sciences. Statistical analysis Each experiment was performed at least three times. Data represent mean±s.d. Student’s t -tests were used to compare all samples. Statistically significant differences are shown as follows: * P <0.05, ** P <0.01, *** P <0.001. Accession codes. Microarray and ChIP-seq data have been deposited at Gene Expression Omnibus under accession number GSE66027 . How to cite this article: Liu, P. et al . Histone deacetylation promotes mouse neural induction by restricting Nodal-dependent mesendoderm fate. Nat. Commun . 6:6830 doi: 10.1038/ncomms7830 (2015).